High-mobility hydrogenated polycrystalline In2O3(In2O3:H) thin-film transistors Oxide semiconductors have been extensively studied as active channel layers of thin-film transistors (TFTs) for electronic applications. However, the field-effect mobility ( μ FE ) of oxide TFTs is not sufficiently high to compete with that of low-temperature-processed polycrystalline-Si TFTs (50–100 cm 2 V −1 s −1 ). Here, we propose a simple process to obtain high-performance TFTs, namely hydrogenated polycrystalline In 2 O 3 (In 2 O 3 :H) TFTs grown via the low-temperature solid-phase crystallization (SPC) process. In 2 O 3 :H TFTs fabricated at 300 °C exhibit superior switching properties with µ FE = 139.2 cm 2 V −1 s −1 , a subthreshold swing of 0.19 Vdec −1 , and a threshold voltage of 0.2 V. The hydrogen introduced during sputter deposition plays an important role in enlarging the grain size and decreasing the subgap defects in SPC-prepared In 2 O 3 :H. The proposed method does not require any additional expensive equipment and/or change in the conventional oxide TFT fabrication process. We believe these SPC-grown In 2 O 3 :H TFTs have a great potential for use in future transparent or flexible electronics applications. Wide-bandgap oxide semiconductors (OSs) have been extensively studied as active channel layers of thin-film transistors (TFTs) for next-generation flat-panel displays [1] , [2] , nonvolatile memories [3] , inverters [4] , various sensors [5] , [6] , Schottky devices [7] , [8] , and so on. Among OSs, amorphous In–Ga–Zn–O (a-IGZO) TFTs have now become the backplane standard for active-matrix liquid-crystal displays (AMLCDs) and active-matrix organic light-emitting diode (AMOLED) displays because of their reasonable field-effect mobility ( μ FE ) of over 10 cm 2 V −1 s −1 , extremely low leakage current, low process temperature (<350 °C), and large-area scalability [9] , [10] . Although the μ FE value of a-IGZO TFTs is more than ten times higher than that of hydrogenated amorphous Si (a-Si:H) TFTs (<1 cm 2 V −1 s −1 ), it is not sufficiently high to compete with that of low-temperature-processed polycrystalline-Si (LTPS) TFTs (50–100 cm 2 V −1 s −1 ) [11] . The main disadvantages of LTPS TFTs are a relatively high process temperature (450–550 °C) and an expensive crystallization process. The high μ FE values of OS TFTs mean these devices could be used in fields that have been dominated by LTPS TFTs and in transparent and flexible devices that are incompatible with Si. Numerous types of approaches to enhance the μ FE value of OS TFTs have been investigated, including cation composition [12] , [13] , multiple channel structures [14] , [15] , dual-gate architecture [16] , [17] , metal capping layer structures [18] , [19] , post treatment [20] , [21] , and their combination. Among these, cation composition control is the most promising method. It requires no extra complex process for integrating OS TFTs. In-rich OSs have been studied extensively. The large spatial spread of the In 5 s orbital with a large overlap can provide a facile electron transport path with a low electron effective mass [22] . However, undoped In 2 O 3 films exhibit a high background electron concentration (10 19 –10 21 cm −3 ) [23] , [24] , which is attributable to the presence of native defects, such as oxygen vacancies, making it difficult to control the threshold voltage of the TFTs [25] , [26] . To suppress the carrier concentration in In 2 O 3 , elements such as Ga, Hf, Si, Al, and W were added, which have large bond dissociation energies with oxygen [12] . Many AOS TFTs have been explored with multicomponent oxide semiconductors, such as In–W–Zn–O [27] , Al–In–Sn–Zn–O [28] , and In–Ga–Zn–Sn–O [29] . However, multicomponent oxides complicate the composition control of the deposited film. Moreover, multimetal cations cause potential fluctuation near the conduction band minimum, which might hinder electron transport [30] . Recently, crystalline OSs have been proposed to enhance the carrier mobility because the disorder-induced subgap states can be suppressed via lattice ordering. Yang et al. reported a μ FE value of 60.7 cm 2 V −1 s −1 for a TFT obtained using polycrystalline In–Ga–O annealed at 700 °C [31] . Although high annealing temperatures result in better electrical properties of the oxide active channel layer, such high temperatures are unsuitable for device application on glass or plastic substrates. Our group reported a μ FE value of 50.6 cm 2 V −1 s −1 for a TFT obtained using hydrogenated polycrystalline In–Ga–O formed via solid-phase crystallization (SPC) at 300 °C [32] . This study proposes a simple material and a simple process to obtain high-performance TFTs, namely hydrogenated polycrystalline In 2 O 3 (In 2 O 3 :H) TFTs grown via the low-temperature SPC process. In 2 O 3 :H TFTs fabricated at 300 °C exhibit superior switching properties with µ FE = 139.2 cm 2 V −1 s −1 , a subthreshold swing ( SS ) of 0.19 V dec −1 , and a threshold voltage ( V th ) of 0.2 V. The hydrogen introduced during sputter deposition plays an important role in enlarging the grain size and decreasing the subgap defects in SPC-prepared In 2 O 3 :H. The proposed method has great potential for future transparent or flexible electronics applications. Structural properties of the In 2 O 3 and In 2 O 3 :H films Figures 1 a, b show the XRD patterns of the 50-nm-thick In 2 O 3 and In 2 O 3 :H films deposited at various R [H 2 ] values and at a constant R [O 2 ] of 1%. For the as-deposited films (Fig. 1a ), the In 2 O 3 film without H 2 introduction exhibited a clear crystalline nature with the (222) preferred orientation of the cubic bixbyite In 2 O 3 crystal. There was no noticeable peak for the In 2 O 3 :H films deposited at R [H 2 ] values of 3 and 5%. This result indicates that H 2 addition suppresses the growth of crystallites during deposition. After annealing at 250 °C in nitrogen for 1 h, the amorphous phase of In 2 O 3 :H changed to the crystalline one with the (222) preferred orientation. The angles of the diffracted peaks are in good agreement with the In 2 O 3 powder data (ICSD code: 14388). Moreover, the crystallized films exhibited smaller full-width at half-maximum values of the (222) reflection than the film deposited without hydrogen introduction, indicating larger crystallite sizes and smaller strains in the In 2 O 3 :H films. Fig. 1: Structural properties of the In 2 O 3 and In 2 O 3 :H films. XRD patterns of the In 2 O 3 and In 2 O 3 :H films deposited at different R [H 2 ] values and at a constant R [O 2 ] value of 1% a before and b after annealing at 250 °C in N 2 . EBSD images of the In 2 O 3 and In 2 O 3 :H films deposited at different R [H 2 ] values c – e before and f – h after annealing at 250 °C in N 2 . Area fraction of each grain size obtained from the In 2 O 3 and In 2 O 3 :H films deposited at different R [H 2 ] values i before and j after annealing at 250 °C in N 2 . 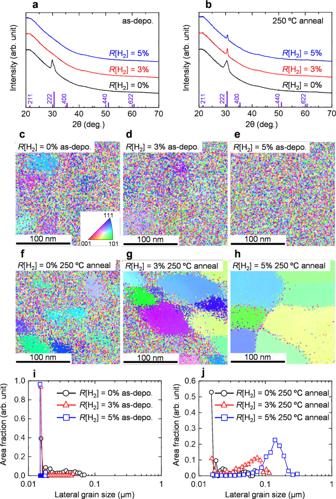Fig. 1: Structural properties of the In2O3and In2O3:H films. XRD patterns of the In2O3and In2O3:H films deposited at differentR[H2] values and at a constantR[O2] value of 1%abefore andbafter annealing at 250 °C in N2. EBSD images of the In2O3and In2O3:H films deposited at differentR[H2] valuesc–ebefore andf–hafter annealing at 250 °C in N2. Area fraction of each grain size obtained from the In2O3and In2O3:H films deposited at differentR[H2] valuesibefore andjafter annealing at 250 °C in N2. Full size image Figure 1 c– h depict the EBSD images along the normal direction for the In 2 O 3 and In 2 O 3 :H films with and without annealing at 250 °C in nitrogen. For the as-deposited films (Fig. 1c–e ), a randomly oriented small grain structure embedded in the amorphous matrix can be observed in the In 2 O 3 film without H 2 introduction. The grain structure disappeared upon increasing the R [H 2 ] value to 5%. In contrast, a huge grain structure appeared for In 2 O 3 :H deposited at R [H 2 ] = 5% after annealing at 250 °C (Fig. 1h ), indicating SPC occurrence. This is consistent with the results of the XRD analysis shown in Fig. 1a, b . The corresponding area fractions of each lateral grain size are shown in Fig. 1i, j . The detected minimum grain size is around 15 nm, which is limited by the electron beam size of the EBSD measurements. For the as-deposited films (Fig. 1i ), all films showed the maximum area fraction for a grain size of 15 nm; however, a small proportion of the area fraction with a grain size of ~70 nm was detected in the In 2 O 3 film, indicating nuclei in the as-deposited film. After annealing at 250 °C (Fig. 1j ), the peak of the area fraction shifted toward a larger grain size as R [H 2 ] increased, and the In 2 O 3 :H film deposited at R [H 2 ] = 5% showed a maximum area fraction of 23% at a grain size of 140 nm. Furthermore, as R [H 2 ] increased from 0 to 5%, the area fraction of the minimum grain size below 15 nm significantly decreased, and only a few small grains were in between the large grains, as shown in Fig. 1h . Similar results were observed for films annealed at 250 °C in ambient air (shown in Supplementary Fig. 1 ). The EBSD results show that the nuclei density in the as-deposited film was suppressed by introducing hydrogen during sputtering. Because of the reduction in the nuclei density in the initial In 2 O 3 :H film, the grain size of the In 2 O 3 :H film could be enlarged through SPC. Thus, the XRD and EBSD results indicate that controlling the crystallinity and nuclei density in the as-deposited film are key factors to achieve high-quality In 2 O 3 :H films. 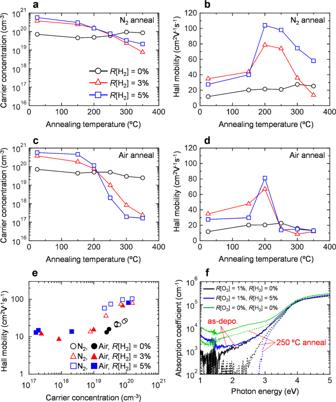Fig. 2: Electrical and optical properties of the In2O3and In2O3:H films. aNeandbµHof In2O3and In2O3:H deposited at differentR[H2] values as a function of the annealing temperature in N2.cNeanddµHof In2O3and In2O3:H deposited at differentR[H2] values as a function of the annealing temperature in ambient air.eThe relationship betweenµHandNefor the films annealed atTann> 200 °C in N2and ambient air.fOptical absorption spectra of the 50-nm-thick In2O3and In2O3:H films deposited at differentR[H2] values before and after annealing at 250 °C in ambient air. In2O3films deposited without oxygen and hydrogen are also shown for comparison. Electrical and optical properties of the In 2 O 3 and In 2 O 3 :H films Figure 2a–d show the carrier concentration ( N e ) and Hall mobility ( µ H ) of the 50-nm-thick In 2 O 3 and In 2 O 3 :H films deposited at various R [H 2 ] values as a function of the annealing temperature ( T ann ). Koida et al. reported that both the N e and µ H of the SPC-prepared In 2 O 3 :H films decrease dramatically for the films annealed in vacuum at T ann > 400 °C due to the desorption of the H 2 O and H 2 gases from the films and additional microscopic defects inside the grains [33] . The electrical properties of OSs are strongly affected by the annealing atmosphere [34] ; thus, annealing treatments at temperatures ranging from 150 to 350 °C in nitrogen and ambient air were examined. For the as-deposited films, N e increased from 7.1 × 10 19 to 5.7 × 10 20 cm −3 upon increasing R [H 2 ] from 0 to 5%, as shown in Fig. 2a . Since hydrogen acts as a shallow donor in In 2 O 3 [35] , the increase in the N e of the as-deposited In 2 O 3 :H film upon increasing R [H 2 ] is attributable to hydrogen doping effects. The In 2 O 3 film deposited without hydrogen introduction exhibited an almost constant N e value over the whole range of investigated T ann values irrespective of the annealing atmosphere, as shown in Fig. 2 a, c . In contrast, there was a strong dependence of N e on the annealing atmosphere for the In 2 O 3 :H films. The N e of the In 2 O 3 :H film annealed in N 2 gradually decreased with increasing T ann (Fig. 2a ), whereas the N e of the In 2 O 3 :H film annealed in air rapidly decreased for T ann > 200 °C (Fig. 2c ). In addition, the N e reduction was remarkable in the In 2 O 3 :H film deposited at a higher R [H 2 ] value. As a result, an appropriate N e value of 2.0 × 10 17 cm −3 for TFT fabrication was obtained at T ann = 300 °C for the In 2 O 3 :H film deposited at R [H 2 ] = 5%; this N e value is over two orders of magnitude lower than that of the In 2 O 3 film deposited without hydrogen introduction (3.0 × 10 19 cm −3 ). Such a large decrease in the N e value of the In 2 O 3 :H films has not been reported before. Although adding H 2 induced the formation of free carriers in the as-deposited films, the N e of the films could be reduced via the relatively low-temperature SPC process and became comparable to that of single-crystalline epitaxial In 2 O 3 films deposited at 650 °C (~1 × 10 17 cm −3 ) [36] . Fig. 2: Electrical and optical properties of the In 2 O 3 and In 2 O 3 :H films. a N e and b µ H of In 2 O 3 and In 2 O 3 :H deposited at different R [H 2 ] values as a function of the annealing temperature in N 2 . c N e and d µ H of In 2 O 3 and In 2 O 3 :H deposited at different R [H 2 ] values as a function of the annealing temperature in ambient air. e The relationship between µ H and N e for the films annealed at T ann > 200 °C in N 2 and ambient air. f Optical absorption spectra of the 50-nm-thick In 2 O 3 and In 2 O 3 :H films deposited at different R [H 2 ] values before and after annealing at 250 °C in ambient air. In 2 O 3 films deposited without oxygen and hydrogen are also shown for comparison. Full size image Regarding the Hall mobility of the films, In 2 O 3 without hydrogen introduction exhibited an almost constant µ H value over the entire range of investigated T ann values irrespective of the annealing atmosphere, as shown in Fig. 2b, c . Upon annealing in N 2 at T ann = 200 °C, the µ H of In 2 O 3 :H increased to 78.6 cm 2 V −1 s −1 at R [H 2 ] = 3% and 104.0 cm 2 V −1 s −1 at R [H 2 ] = 5%, indicating that the SPC started at a T ann value between 150 and 200 °C. Furthermore, the increased µ H is attributable to the increased grain size, as shown in Fig. 1f–h . As T ann increased, the µ H of In 2 O 3 :H gradually decreased (Fig. 2b ). Upon annealing in air (Fig. 2d ), the maximum µ H of In 2 O 3 :H decreased slightly to 67.1 cm 2 V −1 s −1 at R [H 2 ] = 3% and 81.2 cm 2 V −1 s −1 at R [H 2 ] = 5%, and the decrease in µ H for T ann > 250 °C was confirmed. To understand the transport properties of the In 2 O 3 :H films after SPC, the relationship between µ H and N e for the films annealed in the range of temperatures between 200 °C and 350 °C in N 2 and ambient air was summarized, as shown in Fig. 2e . The N e of the In 2 O 3 :H film could be controlled by up to three orders of magnitude. Moreover, for the N e range between 10 19 and 10 20 cm −3 , µ H increases with increasing R [H 2 ], which is attributable to the suppression of grain boundary scattering due to the increasing grain size. For all the films, µ H increased with increasing N e . In general, the grain boundaries have a small impact on µ H in transparent conductive oxides with high N e (>10 20 cm −3 ) because electrons can tunnel through the narrow width (<1 nm) of the grain barriers at high N e values (>10 20 cm −3 ). However, grain boundary scattering is a dominant factor that limits the µ H in films with lower N e [37] . Thus, the observed decrease in µ H with decreasing N e (Fig. 2e ) is due to grain boundary scattering. Although the µ H of In 2 O 3 :H decreased for N e < 10 19 cm −3 , carriers (with number in the range of 10 19 –10 20 cm −3 ) will be generated at the In 2 O 3 :H/gate insulator interface of the TFTs when applying a voltage to the gate [15] ; thus, a high µ FE can be expected in In 2 O 3 :H TFTs. Figure 2f shows the optical absorption ( α ) spectra of the In 2 O 3 and In 2 O 3 :H films before and after annealing at 250 °C in ambient air. The green line represents the In 2 O 3 film deposited without oxygen and hydrogen (only Ar gas), which is shown for comparison. The spectral features that arise as the photon energy exceeds 2.9 eV are due to the absorption associated with the interband transition in In 2 O 3 , whereas the features that arise when the photon energy is below 1.5 eV are due to free carrier absorption. The absorption in the subgap region (<2.9 eV) dropped as R [O 2 ] increased from 0 to 1%, suggesting that oxygen deficiencies, which give rise to subgap defects, are compensated when sputtering in an oxidizing atmosphere. When hydrogen is added during sputter deposition, the absorption is enhanced in the subgap region for the as-deposited films, especially in the photon energy region below 1.5 eV, indicating that free electron absorption is increased due to the hydrogen doping effect. On the other hand, after annealing at 250 °C in ambient air (dashed line), the absorption across the subgap of the In 2 O 3 :H film decreased significantly and was lower than that of the In 2 O 3 film. Since subgap defects are generated from native defects, such as oxygen vacancies, as described above, it can be inferred that oxygen vacancies were efficiently reduced in In 2 O 3 :H via SPC in ambient air. This result is consistent with the Hall effect measurements, where it was found that N e decreased from 5.7 × 10 20 to 2.0 × 10 18 cm −3 upon annealing in air at 250 °C, as shown in Fig. 2c . The structural, electrical, and optical properties of the In 2 O 3 :H films show that the hydrogen introduced during sputter deposition plays an important role in enlarging the grain size and decreasing the subgap defects after SPC, increasing µ H and decreasing N e . However, a more detailed study will be necessary to carry out quantitative evaluations of the carrier generation and scattering in the SPC-prepared In 2 O 3 :H films. 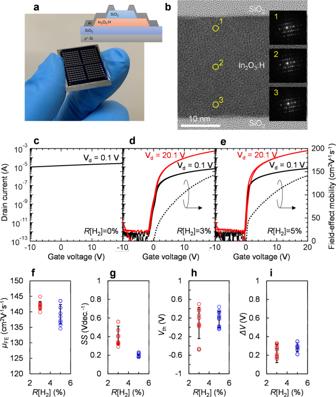Fig. 3: In2O3:H TFT characteristics. aPhotograph and schematic cross-sectional view of the SPC-prepared In2O3:H TFTs.bHRTEM image and corresponding SAED pattern of the active layer of the TFT with In2O3:H channel deposited atR[H2] = 5%.c–eTypical transfer characteristics of the TFTs with In2O3and In2O3:H channels deposited at variousR[H2] values. Variations offµFE,gSS,hVth, andiΔVevaluated from ten TFTs. In 2 O 3 :H TFT characteristics Figure 3a shows the picture and schematic cross-sectional view of the fabricated In 2 O 3 :H TFT. All TFTs were fabricated using annealing in ambient air at 300 °C. Figure 3c–e show typical transfer characteristics of the TFTs with In 2 O 3 and In 2 O 3 :H channels deposited at various R [H 2 ] values. The variations of µ FE , subthreshold swing (SS), threshold voltage ( V th ), and hysteresis (Δ V ) were evaluated from ten TFTs on the same substrate. The µ FE was calculated from the linear transfer characteristics as µ FE = Lg m /(WC ox V ds ) at V ds = 0.1 V, where g m is the transconductance, C ox is the oxide capacitance of the gate insulator, and V ds is the drain voltage. V th was defined by gate voltage ( V gs ) at drain current ( I ds ) of 1 nA, and SS was extracted from V gs , which required an increase in the I ds from 10 to 100 pA. The In 2 O 3 TFT without H 2 introduction (Fig. 3c ) did not exhibit any switching (conductive behavior). By contrast, the In 2 O 3 :H TFT deposited at R [H 2 ] = 5% exhibited a switching with an extremely high µ FE of 139.2 cm 2 V −1 s −1 , a SS of 0.19 V dec −1 , a V th of 0.2 V, and a Δ V of 0.3 V as shown in Table 1 . The TFT with In 2 O 3 :H deposited at R [H 2 ] = 5% showed a slightly small SS value (0.19 V dec −1 ) compared with that of the TFT with In 2 O 3 :H deposited at R [H 2 ] = 3% (0.41 V dec −1 ). The subgap density of states ( D sg ) at the Fermi level was calculated as SS = d V gs /dlog I ds = ln10 k B T / e (1 + eD sg / C ox ), where k B is Boltzmann’s constant and e is the elementary electric charge [10] . The D sg decreased from 1.3 × 10 12 to 4.7 × 10 11 cm −2 eV −1 by increasing the R [H 2 ] value from 3 to 5%. This result suggests that the disorder-originated subgap defect states near the conduction band minimum can be reduced in the In 2 O 3 :H channel deposited at R [H 2 ] = 5%, which is confirmed by the optical measurements of the films shown in Fig. 2f . Fig. 3: In 2 O 3 :H TFT characteristics. a Photograph and schematic cross-sectional view of the SPC-prepared In 2 O 3 :H TFTs. b HRTEM image and corresponding SAED pattern of the active layer of the TFT with In 2 O 3 :H channel deposited at R [H 2 ] = 5%. c – e Typical transfer characteristics of the TFTs with In 2 O 3 and In 2 O 3 :H channels deposited at various R [H 2 ] values. Variations of f µ FE , g SS, h V th , and i Δ V evaluated from ten TFTs. Full size image Table 1 Summary of the TFT properties. Full size table The resulting transfer performance of the SPC-prepared In 2 O 3 :H TFT ( R [H 2 ] = 5%) was superior to that of previously reported oxide-based TFTs [38] . Although the µ H of the In 2 O 3 :H ( R [H 2 ] = 5%) films decreased to 14.9 cm 2 V −1 s −1 with N e of 2.0 × 10 17 cm −3 by annealing at 300 °C as shown in Fig. 2c , extremely high µ FE was obtained from the TFTs because a large number of carriers (10 19 –10 20 cm −3 ) was generated at the In 2 O 3 :H/gate insulator interface when applying a voltage to the gate, which allows electrons to tunnel through the narrow width (<1 nm) of the grain barriers at high N e values. The high µ FE and steep SS of the In 2 O 3 :H TFTs can be attributed to the high crystallinity of In 2 O 3 :H, especially near the In 2 O 3 :H/SiO 2 gate insulator interface. Figure 3b shows a cross-sectional conventional bright-field HRTEM image and selective area electron diffraction (SAED) pattern obtained from the SPC-prepared In 2 O 3 :H TFT ( R [H 2 ] = 5%). A clear lattice image was observed over the entire thickness of the In 2 O 3 :H channel. Moreover, there was a single crystal-like diffraction pattern in the SAED pattern, even in the thin layers, roughly at a distance of 5 nm from the SiO 2 gate insulator without detectable diffuse ring patterns, which would be attributable to an amorphous phase. This observation explains the high µ FE of 139.2 cm 2 V −1 s −1 in the In 2 O 3 :H TFTs, which is comparable to the µ H of epitaxial single-crystal In 2 O 3 films (~160 cm 2 V −1 s −1 ) [39] . In addition, although In 2 O 3 :H is a polycrystalline film, the standard deviations ( σ ) of µ FE , SS , V th , and Δ V of the In 2 O 3 :H TFT ( R [H 2 ] = 5%) were 3.0 cm 2 V −1 s −1 , 0.02 V dec −1 , 0.2 V, and 0.1 V, respectively, indicating high uniformity of the TFT characteristics (shown in Fig. 3f–i and Supplementary Fig. 2 ). To investigate the reliability of the SPC-prepared In 2 O 3 :H TFT ( R [H 2 ] = 5%), positive-bias stress (PBS) and negative-bias stress (NBS) tests were carried out under a humidity of 50%. The gate stress voltages for the PBS and NBS were +20 and −20 V, respectively. 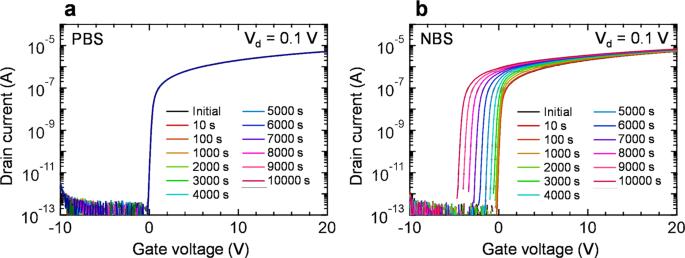Fig. 4: Reliability of the In2O3:H TFT. Changes in the transfer characteristics of the In2O3:H (R[H2] = 5%) TFT during theaPBS andbNBS tests. TheVgsvalues under the PBS and NBS tests were +20 and −20 V, respectively. Figure 4 a, b show the changes in the transfer characteristics of the In 2 O 3 :H TFT during the PBS and NBS tests. The In 2 O 3 :H TFT showed no significant positive shift in V th (only +0.02 V) under the PBS test, indicating the negligible interfacial trap states in the In 2 O 3 :H/SiO 2 gate insulator interface as well as the high quality of the In 2 O 3 :H channel layer. In contrast, a large V th shift of –4.4 V was observed for the NBS test, as shown in Fig. 4b . Furthermore, the V th shift became more significant when the NBS test was conducted at a higher humidity of 70% (shown in Supplementary Fig. 3 ). Water molecules are coupled to the backchannel of the IGZO TFTs, and excess electrons are donated to the channel under NBS, resulting in a negative V th shift [40] , [41] . Applying a passivation layer to the TFTs is effective in minimizing the influence of the atmospheric environment; however, hydrogen can diffuse into the channel through the passivation layer and increase the N e of the channel [42] . Although the SiO 2 passive layer was applied to the SPC-grown In 2 O 3 :H TFT, as shown in Fig. 3a , its protection ability was insufficient because the SiO 2 film was deposited via sputtering at RT. Hence, it is believed that the reliability of In 2 O 3 :H TFTs can be improved by selecting the appropriate passivation layer, such as SiN, Al 2 O 3 , or Y 2 O 3 . Fig. 4: Reliability of the In 2 O 3 :H TFT. Changes in the transfer characteristics of the In 2 O 3 :H ( R [H 2 ] = 5%) TFT during the a PBS and b NBS tests. The V gs values under the PBS and NBS tests were +20 and −20 V, respectively. Full size image In this study, we demonstrate the high-performance polycrystalline In 2 O 3 :H TFTs using a low-temperature SPC process. To ensure the amorphous state of the as-deposited In 2 O 3 :H film, a moderate amount of H 2 was introduced into the sputtering system during the In 2 O 3 :H deposition. The as-deposited amorphous In 2 O 3 :H film converted into a polycrystalline In 2 O 3 :H film with a grain size of around 140 nm via low-temperature SPC (at a temperature below 200 °C). As a result, a high µ H of 104.0 cm 2 V −1 s −1 was obtained for the In 2 O 3 :H film. This µ H value is five times higher than that of the In 2 O 3 film without H 2 introduction during sputtering. Furthermore, the N e of the SPC-grown In 2 O 3 :H film decreased significantly to 2.0 × 10 17 cm −3 after annealing at 300 °C in ambient air; this N e value is two orders of magnitude lower than that of the In 2 O 3 film without H 2 introduction. Thus, introducing hydrogen during sputtering followed by annealing in ambient air is an effective method for improving both the crystallinity and the N e value of In 2 O 3 :H films. The obtained In 2 O 3 :H film was employed as the channel of a TFT, and the resulting In 2 O 3 :H TFT exhibits an extremely high µ FE of 139.2 cm 2 V −1 s −1 , an appropriate V th of 0.2 V, and a small SS of 0.19 V dec −1 . HRTEM analysis of the TFT revealed the high crystallinity of cubic bixbyite near the In 2 O 3 :H/SiO 2 gate dielectric interface, which contributed to the high µ FE of the TFT. The proposed method does not require any additional expensive equipment and/or change in the conventional oxide TFT fabrication process. Moreover, composition control of binary In 2 O 3 films is easier than that of ternary and quaternary semiconductors. We believe that these SPC-grown In 2 O 3 :H TFTs are promising candidates for use in future transparent or flexible electronics applications. Fabrication of In 2 O 3 :H TFTs In 2 O 3 :H TFTs were fabricated on a heavily doped p -type Si substrate with a 100-nm-thick thermally grown SiO 2 . The doped p -type Si substrate and the SiO 2 were used as the gate electrode and the gate insulator. The 30-nm-thick In 2 O 3 and In 2 O 3 :H channels were deposited via pulsed direct-current (DC) magnetron sputtering without substrate heating from a ceramic In 2 O 3 target using a mixture of Ar, O 2 , and H 2 gases. The O 2 and H 2 gas flow ratios are R [O 2 ] = O 2 /(Ar + O 2 + H 2 ) and R [H 2 ] = H 2 /(Ar + O 2 + H 2 ), respectively. For the Ar + O 2 -sputtered In 2 O 3 film, R [O 2 ] was set to 1% without H 2 introduction. For the Ar + O 2 + H 2 -sputtered In 2 O 3 film (In 2 O 3 :H), R [H 2 ] varied from 3 to 5%, whereas R [O 2 ] was fixed at 1%. The deposition pressure and DC power were maintained at 0.6 Pa and 50 W, respectively. The base pressure before gas introduction was below 6 × 10 −5 Pa. The In 2 O 3 and In 2 O 3 :H films were then annealed in ambient air at 300 °C for 1 h. After annealing, a 100-nm-thick SiO 2 film was deposited via reactive sputtering without substrate heating. This film served as a passive layer. Subsequently, Al source/drain electrodes were deposited via sputtering. Finally, In 2 O 3 and In 2 O 3 :H TFTs were annealed at 250 °C in ambient air for 1 h. The In 2 O 3 , SiO 2 , and Al films were deposited through a shadow mask. Both the channel length and the width were 300 µm. Characterization of the In 2 O 3 :H films and TFTs Structural, electrical, and optical measurements were conducted on the 50-nm-thick In 2 O 3 and In 2 O 3 :H films deposited on a synthetic quartz substrate. The films’ structural changes were evaluated through X-ray diffraction (XRD) (Philips corp., X’pert) with CuK α radiation and electron backscattering diffraction (EBSD) (EDAX-TSL Hikari High Speed EBSD Detector). The films’ carrier concentrations ( N e ) and Hall mobility ( µ H ) were determined via Hall effect measurements (Accent, HL5500PC) using the van der Pauw geometry at room temperature (RT). The films’ optical properties were measured via spectrophotometry (Hitachi, U-4100). The current–voltage characteristics were measured using a semiconductor parameter analyzer (Keysight, E5270B) at RT in the dark. High-resolution transmission electron microscopy (HRTEM) (JEOL, JSM-7001F) analysis was also conducted to observe the microstructure of the In 2 O 3 :H channel in the TFTs.